APC/C-Cdh1 coordinates neurogenesis and cortical size during development The morphology of the adult brain is the result of a delicate balance between neural progenitor proliferation and the initiation of neurogenesis in the embryonic period. Here we assessed whether the anaphase-promoting complex/cyclosome (APC/C) cofactor, Cdh1—which regulates mitosis exit and G1-phase length in dividing cells—regulates neurogenesis in vivo . We use an embryo-restricted Cdh1 knockout mouse model and show that functional APC/C-Cdh1 ubiquitin ligase activity is required for both terminal differentiation of cortical neurons in vitro and neurogenesis in vivo . Further, genetic ablation of Cdh1 impairs the ability of APC/C to promote neurogenesis by delaying the exit of the progenitor cells from the cell cycle. This causes replicative stress and p53-mediated apoptotic death resulting in decreased number of cortical neurons and cortex size. These results demonstrate that APC/C-Cdh1 coordinates cortical neurogenesis and size, thus posing Cdh1 in the molecular pathogenesis of congenital neurodevelopmental disorders, such as microcephaly. The morphology and size of the adult brain strictly depend on the number of neurons that are generated from their progenitor cells during the embryonic period [1] . To ensure that the adequate source of future neurons is timely produced, an intense proliferative activity takes place at the ventricular (VZ) and subventricular (SVZ) zones lining the cerebral ventricles [2] , [3] . In the very early stages of cerebral cortex development, the progenitor cells must divide symmetrically; however, in later stages of development, these neural progenitor cells undergo asymmetric divisions, thus allowing self-renewal and production of either neurons or intermediate progenitor cells [4] , [5] . The latter cells further undergo symmetric, differentiating divisions, to increase the number of neurons, a process that persists until the proliferative cell pool is exhausted [4] , [5] , [6] . Thus, the structure of the brain is the result of a delicate and timely controlled balance between the symmetric divisions to maintain the progenitor cell pool, and the asymmetric divisions to generate a newly differentiated neuron [3] , [4] , [6] . Neurogenesis is a complex process that relies on an as yet unknown molecular switch that tightly coordinates the cell cycle exit with the start of the differentiation process [7] , [8] , [9] , [10] . Recent observations suggest that the cell cycle length is a key factor that determines the balance between the maintenance of progenitor cells and neuronal differentiation [10] . In fact, it has been shown that neurogenesis in the cerebral cortex is stimulated by lengthening the G1 phase [1] , [11] , [12] and delayed by shortening it [13] , [14] ; however, the molecular mechanism that coordinates this process during embryogenesis is unknown. The anaphase-promoting complex/cyclosome (APC/C) is a multisubunit E3 ubiquitin ligase that, by targeting securin, mitotic cyclins and other substrates for proteasomal degradation [15] , regulates the progression from metaphase to anaphase, exit from mitosis and quiescence maintenance [16] . For full functional activity, APC/C requires to be bound to either Cdc20 or Cdh1 cofactors [17] , [18] , [19] . In early mitosis, cyclin–cyclin-dependent kinase (Cdk) complexes phosphorylate several subunits of the APC/C, which bind to Cdc20 leading to the initiation of anaphase [20] . In contrast, during S phase, G2 phase and early mitosis, cyclin–Cdk complexes phosphorylate Cdh1, inhibiting its binding to APC/C [21] , [22] . During late mitosis, cyclin–Cdk complexes are inactivated, and phosphatases are activated, thus dephosphorylating Cdh1 that binds to, and activates, APC/C [23] , [24] . Accordingly, while APC/C-Cdc20 dictates mitotic exit, APC/C-Cdh1 maintains cells in G1 phase [15] , [16] , [23] , [24] . Given its critical role in determining the G1-phase length, we sought to investigate whether APC/C-Cdh1 activity would be responsible for the switch from progenitor cells cycling to neurogenesis in the cerebral cortex. By using Sox2-Cre conditional Cdh1-knockout mice [25] , here we show that functional APC/C-Cdh1 activity is necessary to couple the progenitor cell cycle exit with neuronal differentiation. Further, we show that Cdh1 loss, which shortens G1 phase and extends S phase, causes replicative stress leading to p53-mediated death of neural progenitor cells and reduction of the cortical size. These findings demonstrate that Cdh1 is required for proper cortical neurogenesis, which has important implications in the control of mammalian brain size and the pathogenesis of congenital neurodevelopmental disorders, such as microcephaly (MCPH). APC/C-Cdh1 supports neuronal differentiation and survival To study the possible role of APC/C-Cdh1 in neuronal differentiation, we first established an in vitro model of progressive differentiation of embryonic day 14.5 (E14.5) cells of the mouse brain cortex. As shown in Fig. 1a , cells profusely expressed Cdh1 throughout the 9-day incubation period, showing a progressive increase in its electrophoretic mobility. Map2—a neuronal-specific marker—was absent up to day 2, and then gradually accumulated with an inverse pattern to that of the F-box protein, S-phase kinase-associated protein 2 (Skp2), a substrate of APC/C-Cdh1 (refs 26 , 27 ). In turn, the Cdk inhibitor p27, abundantly and progressively accumulated as from day 2 in culture ( Fig. 1a ). Flow cytometric analyses of these cells revealed a progressive decline in bromodeoxyuridine (BrdU) incorporation ( Supplementary Fig. S1A ) and a decrease in cell cycle activity, as judged by the increased G0/G1 phase and the decrease in S and G2/M phases observed during the first 2 days in culture ( Supplementary Fig. S1B ). Together, these data indicate that mouse cortical cells in culture exit the cell cycle leading to a neuronal phenotype. 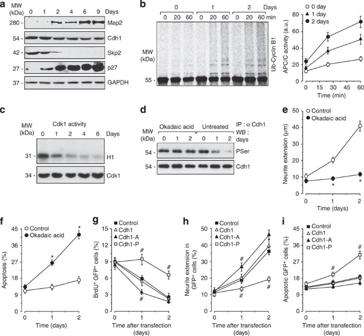Figure 1: Neuronal differentiation and survival is associated to Cdh1 dephosphorylation and APC/C-Cdh1 activation. Mouse cortical cells in culture differentiate to a neuronal phenotype, as showed by western blotting (a). (b) The activity of APC/C-Cdh1 increased during the first 2 days in culture, (c) whereas the activity of cyclin B1-target, Cdk1, rapidly disappeared along the differentiation process. (d) Cdh1 is dephosphorylated as from day 1 in culture, as evidenced by anti-phosphoserine immunoblotting of Cdh1 immunoprecipitates. This effect was prevented by incubation of the cells with the PP2A inhibitor, okadaic acid. Treatment of mouse cortical cells in culture with okadaic acid (e) abolishes the time-dependent increase in neurite extension and (f) triggers apoptotic cell death. At 4 h after plating, cortical cells were transfected with pIRES2-EGFP mammalian expression vector co-expressing the enhanced GFP and either the wild type (Cdh1), phospho-mimetic (Cdh1-P) or non-phosphorylatable (Cdh1-A) forms of Cdh1. Control cells were transfected with empty vector (pIRES2-EGFP). Analysis was performed in transfected (identified by GFP+ fluorescence) cells (day 0: 4–6 h after transfection). Both (g) BrdU incorporation and (h) inhibition of neurite extension are delayed by Cdh1-P but accelerated by Cdh1-A. (I) Cdh1-P, but not by Cdh1-A, induces apoptotic cell death. *P<0.05 versus control.#P<0.05 versus Cdh1 (analysis of variance;n=4 independent culture preparations). Data are expressed as mean±s.e.m. Figure 1: Neuronal differentiation and survival is associated to Cdh1 dephosphorylation and APC/C-Cdh1 activation. Mouse cortical cells in culture differentiate to a neuronal phenotype, as showed by western blotting ( a ). ( b ) The activity of APC/C-Cdh1 increased during the first 2 days in culture, ( c ) whereas the activity of cyclin B1-target, Cdk1, rapidly disappeared along the differentiation process. ( d ) Cdh1 is dephosphorylated as from day 1 in culture, as evidenced by anti-phosphoserine immunoblotting of Cdh1 immunoprecipitates. This effect was prevented by incubation of the cells with the PP2A inhibitor, okadaic acid. Treatment of mouse cortical cells in culture with okadaic acid ( e ) abolishes the time-dependent increase in neurite extension and ( f ) triggers apoptotic cell death. At 4 h after plating, cortical cells were transfected with pIRES2-EGFP mammalian expression vector co-expressing the enhanced GFP and either the wild type (Cdh1), phospho-mimetic (Cdh1-P) or non-phosphorylatable (Cdh1-A) forms of Cdh1. Control cells were transfected with empty vector (pIRES2-EGFP). Analysis was performed in transfected (identified by GFP+ fluorescence) cells (day 0: 4–6 h after transfection). Both ( g ) BrdU incorporation and ( h ) inhibition of neurite extension are delayed by Cdh1-P but accelerated by Cdh1-A. (I) Cdh1-P, but not by Cdh1-A, induces apoptotic cell death. * P <0.05 versus control. # P <0.05 versus Cdh1 (analysis of variance; n =4 independent culture preparations). Data are expressed as mean±s.e.m. Full size image We next assessed whether APC/C-Cdh1 activity mediated the neuronal differentiation process. As shown in Fig. 1b , the activity of APC/C-Cdh1 increased from day 1 to 2, as judged by the ability of APC/C-immunoprecipitated extracts obtained from the brain cortex-cultured cells to ubiquitylate its cognate target, cyclin B1. In contrast, the activity of cyclin B1-target, Cdk1, rapidly disappeared along the differentiation process, as determined by the ability of nuclear extracts to phosphorylate histone H1 ( Fig. 1c ). In Cdh1-immunoprecipitated cell extracts subjected to anti-phosphoserine immunoblotting, we observed Cdh1 spontaneous dephosphorylation as from day 1 in culture ( Fig. 1d ), a phenomenon that was abolished by incubation of the cells with the phosphatase inhibitor, okadaic acid ( Fig. 1d ). These data are compatible with the notion that dephosphorylated Cdh1 is required to support functional APC/C-Cdh1 during in vitro neuronal differentiation. Interestingly, treatment of mouse cortical cells in culture with okadaic acid abolished the time-dependent increase in neurite extension ( Fig. 1e ) and triggered apoptotic cell death ( Fig. 1f ). These results suggest—although do not directly prove—that functional APC/C-Cdh1 is required to promote neuronal differentiation. To further validate this hypothesis, cortical cells at day 0 in culture (4 h after plating) were transfected with either the APC/C inhibitor hEmi1, or with the phospho-mimetic (Cdh1-P) or non-phosphorylatable (Cdh1-A) forms of Cdh1. The APC/C inhibitor hEmi1 significantly increased the percentage of cells in S phase measured by BrdU incorporation ( Supplementary Fig. S1C ) and abolished neurite extension ( Supplementary Fig. S1D ). Interestingly, both BrdU incorporation and inhibition of neurite extension were delayed by Cdh1-P and accelerated by Cdh1-A ( Fig. 1g,h ). Moreover, apoptotic death was increased by both hEmi ( Supplementary Fig. S1E ) and Cdh1-P, but not by Cdh1-A ( Fig. 1i ). Thus, active—dephosphorylated—form of Cdh1 leading to functional APC/C-Cdh1 is able to support neuronal differentiation and survival in vitro . Complete inactivation of Cdh1 leads to embryonic lethality at mid-gestation (E10.5) caused by specific aberrations in the placenta owing to the essential role of this protein in endoreduplication [25] , [28] . These defects were rescued by using a Sox2-Cre transgenic mouse strain that specifically expresses the Cre recombinase in most cells in the developing embryo but not in the placenta [29] . To confirm the essential role of Cdh1 in neuronal differentiation and survival, we next characterized the differentiation process of cortical cells in culture obtained from E14.5 mice with a Sox2-Cre-mediated Cdh1 deficiency [25] . As shown in Fig. 2a , Cdh1 was present at 0–2 days in culture in cortical cells obtained from wild type (Cdh1 +/+ ) and Cdh1 heterozygous (Cdh1 +/− ) mice, but it was absent in cells obtained from Cdh1 −/− mice. Interestingly, an increase in the electrophoretic mobility of Cdh1 was observed from day 1 to 2 in culture both in Cdh1 +/+ and Cdh1 +/− cells, similar to results shown in Fig. 1a . Map2, which appeared at day 2 in culture in Cdh1 +/+ and Cdh1 +/− cells, was not present in Cdh1 −/− cells. Skp2 and cyclin B1 proteins disappeared at day 2 in culture both in Cdh1 +/+ and Cdh1 +/− cells, but not in Cdh1 −/− cells. Moreover, p27 accumulated from day 1 to 2 in culture both in Cdh1 +/+ and Cdh1 +/− cells, but not in Cdh1 −/− cells ( Fig. 2a ). Accordingly, cortical cells cultured from Cdh1 −/− mice maintained their ability to incorporate BrdU up to day 2 ( Fig. 2b ), when they showed a decrease in the G0/G1 phase and an increase in the S and G2/M phases ( Fig. 2c ). This indicate shortening of the G1 phase and enlargement of the S phase in Cdh1-depleted cultured cortical cells, as previously described for human cell lines and mouse embryonic fibroblasts deficient in Cdh1 (refs 25 , 30 , 31 ). It should be noticed that, on day 2 in culture, the proportion of Nestin-positive cells was higher, whereas that of Tuj1-positive cells was lower, in Cdh1 −/− cortical cells when compared with Cdh1 +/+ cells ( Fig. 2d ). In addition, loss of Cdh1 significantly delayed the extension of neurites ( Fig. 2e,f ). The proportion of annexin V-positive/7-Aminoactinomycin D (7-AAD)-negative (apoptotic; Fig. 2g ) and active caspase-3-positive ( Fig. 2h ) cortical cells significantly increased in Cdh1 −/− cultures, but not in Cdh1 +/+ or Cdh1 +/− cultures. Moreover, most of the active caspase-3-positive cells in Cdh1 −/− cultures expressed the neural precursor cell marker Nestin, whereas only 15% expressed the neuronal marker Tuj1 ( Fig. 2i ). These results confirm that Cdh1 is essential for mouse cortical progenitor cells to acquire a fully differentiated phenotype and to survive in culture. 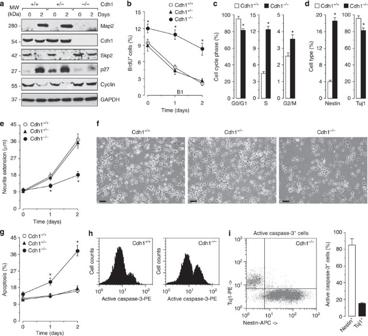Figure 2:Cdh1 deficiency delays cell cycle exit and neuronal differentiation and triggers apoptosisin vitro. Mouse cortical cells in culture were obtained from E14.5 Sox2-Cre conditional Cdh1-knockout mice. (a) Western blot analysis reveals that Cdh1 deficiency (Cdh1−/−) prevents both cell cycle exit and neuronal differentiation, as shown by the accumulation of Skp2 and cyclin B1 and the lack of p27 and Map2 expression. (b) Cortical cells cultured from Cdh1−/−mice maintain their ability to incorporate BrdU and show a (c) decrease in the G0/G-phase and an increase in the S and G2/M phases. (d) After 2 days in culture, the proportion of Nestin-positive cells was higher, whereas that of Tuj1-positive cells was lower, in Cdh1−/−cortical cells when compared with Cdh1+/+cells. (e) Loss of Cdh1 (Cdh1−/−) delayed the extension of neurites of cultured cortical cells. (f) Phase-contrast microscopy of 2 day-cultured mouse cortical cells shows decrease neurite extension and cell number in Cdh1−/−cultures. Scale bar, 50 μm. The proportion of both (g) annexin V-positive/7AAD-negative (apoptotic) and (h) active caspase-3-positive cortical cells significantly increased in cultures obtained from Cdh1−/−embryos, as compared with those obtained from Cdh1+/+or Cdh1+/−embryos. (i) Most (85%) of the apoptotic cells in Cdh1−/−cultures expressed the neural precursor cell marker Nestin. *P<0.05 versus Cdh1+/+(analysis of variance;n=4 independent culture preparations). Data are expressed as mean±s.e.m. Figure 2: Cdh1 deficiency delays cell cycle exit and neuronal differentiation and triggers apoptosis in vitro . Mouse cortical cells in culture were obtained from E14.5 Sox2-Cre conditional Cdh1-knockout mice. ( a ) Western blot analysis reveals that Cdh1 deficiency (Cdh1 −/− ) prevents both cell cycle exit and neuronal differentiation, as shown by the accumulation of Skp2 and cyclin B1 and the lack of p27 and Map2 expression. ( b ) Cortical cells cultured from Cdh1 −/− mice maintain their ability to incorporate BrdU and show a ( c ) decrease in the G0/G-phase and an increase in the S and G2/M phases. ( d ) After 2 days in culture, the proportion of Nestin-positive cells was higher, whereas that of Tuj1-positive cells was lower, in Cdh1 −/− cortical cells when compared with Cdh1 +/+ cells. ( e ) Loss of Cdh1 (Cdh1 −/− ) delayed the extension of neurites of cultured cortical cells. ( f ) Phase-contrast microscopy of 2 day-cultured mouse cortical cells shows decrease neurite extension and cell number in Cdh1 −/− cultures. Scale bar, 50 μm. The proportion of both ( g ) annexin V-positive/7AAD-negative (apoptotic) and ( h ) active caspase-3-positive cortical cells significantly increased in cultures obtained from Cdh1 −/− embryos, as compared with those obtained from Cdh1 +/+ or Cdh1 +/− embryos. ( i ) Most (85%) of the apoptotic cells in Cdh1 −/− cultures expressed the neural precursor cell marker Nestin. * P <0.05 versus Cdh1 +/+ (analysis of variance; n =4 independent culture preparations). Data are expressed as mean±s.e.m. Full size image Loss of Cdh1 triggers replicative stress and apoptotic death To assess whether Cdh1 was involved in cell cycle exit and neuronal differentiation in vivo , we next analysed the brain cortex in Cdh1 −/− E14.5 embryos. Lack of Cdh1 increased mitotic cyclin B1 expression in the cerebral cortex ( Fig. 3a ). Cdh1 deficiency did not significantly alter body weight ( Fig. 3a ) but it decreased (20%) the brain weight ( Fig. 3b ) in comparison with Cdh1 +/+ . However, the brain-to-body-weight ratio ( Supplementary Fig. S2A ) was very similar in heterozygous Cdh1 +/− (bearing both the Cre transgene and the floxed allele) when compared with control Cdh1 +/+ mice. As shown in Fig. 3c , the overall length of the cortex was shorter and unstructured in Cdh1 −/− embryos when compared with the Cdh1 +/+ wild type. This effect was also observed at later stages of development ( Supplementary Fig. S1F,H ). Brain weight ( Supplementary Fig. S1G ) was 27% lower in Cdh1 −/− P0 mice (58.1±2.18 mg) in comparison with age-matched Cdh1 +/+ neonates (80.2±3.16 mg). The developing cortex can be divided into a VZ, SVZ, intermediate zone (IZ) and cortical plate (CP). The VZ is the most apical layer, lining the cerebral ventricles and it constitutes the proliferative region from which all cortical neurons arise [32] . Interestingly, the length of the CP and the IZ were markedly smaller ( Fig. 3c ), but the VZ and SVZ ( Figs 3c and 4a ) were larger in the Cdh1 −/− mice when compared with the Cdh1 +/+ . Since VZ and SVZ contain the neural progenitor niches, we next sought to investigate whether Cdh1 deficiency had any effect on the proportion of neural progenitor cells, and fully differentiated neurons, in these zones. As shown in Fig. 4 , the proportion of Nestin-positive cells ( Fig. 4b,c ) was higher, whereas that of Tuj1- and Map2-positive cells ( Fig. 4a,c ) was lower, in Cdh1 −/− brain sections when compared with sections from Cdh1 +/+ mice, suggesting increased proliferation of neural progenitor cells and decreased neurogenesis in Cdh1-deficient mice. To test this hypothesis further, we analysed the proportion of proliferating cells in the cerebral cortex. As shown in Fig. 5 , both Ki67 ( Fig. 5a ) and BrdU ( Fig. 5b ) fluorescence was dramatically higher in the VZ/SVZ in Cdh1 −/− mice when compared with Cdh1 +/+ mice, indicating increased DNA replication in the mutant brains. It should be noted that the proportion of Tuj1-, Nestin- ( Supplementary Fig. S2B ) and BrdU- ( Supplementary Fig. S2C ) positive cells in brain sections from Cdh1 +/− mice were similar to that found in Cdh1 +/+ mice, ruling out the possible effect of Cre expression on neural progenitor differentiation and proliferation. Together, these results indicate that the lack of Cdh1 extends S-phase length of neural progenitor cells of the VZ/SVZ of the cerebral cortex at the expense of an overall reduction in newly differentiated neurons. 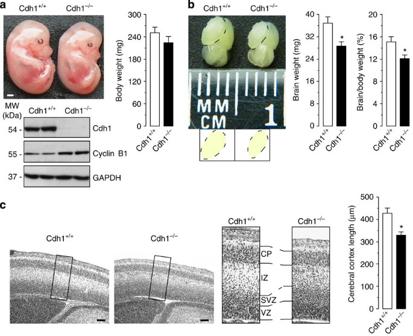Figure 3:Cdh1 deficiency reduces brain size and cerebral cortex lengthin vivo. (a) Cdh1 loss did not modify body size but (b) significantly decreased brain weight in E14.5 mouse embryos. Scale bar, 100 μm. (c) The overall length of the cortex was shorter and unstructured in Cdh1−/−mice when compared with that of Cdh1+/+mice. The length of the intermediate zone (IZ) was smaller, but the ventricular (VZ) and subventricular (SVZ) zones were larger in the Cdh1−/−mice when compared with the Cdh1+/+controls. Scale bar, 100 μm. *P<0.05 versus Cdh1+/+(Student’st-test;n=6 mice). Data are expressed as mean±s.e.m. Figure 3: Cdh1 deficiency reduces brain size and cerebral cortex length in vivo . ( a ) Cdh1 loss did not modify body size but ( b ) significantly decreased brain weight in E14.5 mouse embryos. Scale bar, 100 μm. ( c ) The overall length of the cortex was shorter and unstructured in Cdh1 −/− mice when compared with that of Cdh1 +/+ mice. The length of the intermediate zone (IZ) was smaller, but the ventricular (VZ) and subventricular (SVZ) zones were larger in the Cdh1 −/− mice when compared with the Cdh1 +/+ controls. Scale bar, 100 μm. * P <0.05 versus Cdh1 +/+ (Student’s t -test; n =6 mice). Data are expressed as mean±s.e.m. 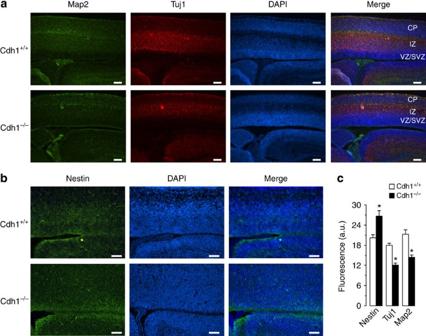Figure 4: Cdh1 deficiency increases neural progenitor population in the VZ and SVZ of the cerebral cortex. (a) Fluorescent photomicrographs of both E14.5 Cdh1+/+and Cdh1−/−cerebral cortex after immunostaining for neuronal differentiation markers (Tuj1: early post-mitotic neurons; Map2: mature post-mitotic neurons). Cdh1 deficiency increases VZ/SVZ length in the brain cortex from E14.5 mice. Scale bar, 100 μm. (b) Fluorescent photomicrographs of both E14.5 Cdh1+/+and Cdh1−/−cerebral cortex after immunostaining for neural progenitor marker, nestin. Scale bar, 50 μm. (c) The proportion of Nestin-positive cells in the VZ/SVZ was higher, whereas that of Tuj1- and Map2-positive cells was lower, in brain sections from Cdh1−/−mice when compared with the corresponding sections of Cdh1+/+mice. *P<0.05 versus Cdh1+/+(Student’st-test;n=4 mice). Data are expressed as mean±s.e.m. Full size image Figure 4: Cdh1 deficiency increases neural progenitor population in the VZ and SVZ of the cerebral cortex. ( a ) Fluorescent photomicrographs of both E14.5 Cdh1 +/+ and Cdh1 −/− cerebral cortex after immunostaining for neuronal differentiation markers (Tuj1: early post-mitotic neurons; Map2: mature post-mitotic neurons). Cdh1 deficiency increases VZ/SVZ length in the brain cortex from E14.5 mice. Scale bar, 100 μm. ( b ) Fluorescent photomicrographs of both E14.5 Cdh1 +/+ and Cdh1 −/− cerebral cortex after immunostaining for neural progenitor marker, nestin. Scale bar, 50 μm. ( c ) The proportion of Nestin-positive cells in the VZ/SVZ was higher, whereas that of Tuj1- and Map2-positive cells was lower, in brain sections from Cdh1 −/− mice when compared with the corresponding sections of Cdh1 +/+ mice. * P <0.05 versus Cdh1 +/+ (Student’s t -test; n =4 mice). Data are expressed as mean±s.e.m. 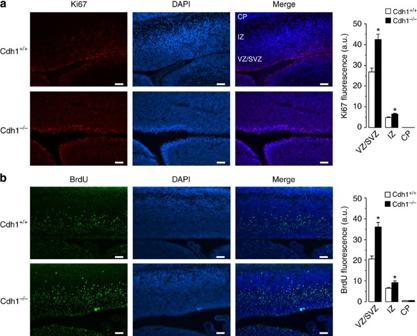Figure 5: Cdh1 deficiency extends proliferation of neural progenitor cells in the VZ and SVZ of the cerebral cortex. Fluorescent photomicrographs of both E14.5 Cdh1+/+and Cdh1−/−cerebral cortex after immunostaining for proliferation markers: (a) Ki67, a cell cycle marker and (b) BrdU, a marker for cells in S phase. Both Ki67 and BrdU fluorescence in the VZ and SVZ was significantly higher in brain sections from Cdh1−/−mice than in the corresponding sections from Cdh1+/+mice. Scale bar, 50 μm. *P<0.05 versus Cdh1+/+(Student’st-test;n=4 mice). Data are expressed as mean±s.e.m. Full size image Figure 5: Cdh1 deficiency extends proliferation of neural progenitor cells in the VZ and SVZ of the cerebral cortex. Fluorescent photomicrographs of both E14.5 Cdh1 +/+ and Cdh1 −/− cerebral cortex after immunostaining for proliferation markers: ( a ) Ki67, a cell cycle marker and ( b ) BrdU, a marker for cells in S phase. Both Ki67 and BrdU fluorescence in the VZ and SVZ was significantly higher in brain sections from Cdh1 −/− mice than in the corresponding sections from Cdh1 +/+ mice. Scale bar, 50 μm. * P <0.05 versus Cdh1 +/+ (Student’s t -test; n =4 mice). Data are expressed as mean±s.e.m. Full size image Our data therefore reveal that the loss of APC/C-Cdh1 activity prevents neural progenitor cells from exiting the cell cycle in vivo , thus confirming the conclusions drawn from the brain cortical cultured cells in vitro ( Fig. 2b,c ). Considering that Cdh1 deficiency causes apoptotic death of cultured neural progenitor cells ( Fig. 2f–i ), we next studied whether this effect occurred in vivo . As depicted in Fig. 6a , Cdh1 loss induced apoptotic cell death as shown by the dramatic increase in the proportion of active caspase-3-positive cells in the VZ/SVZ. To further confirm the progenitor cell nature of the dying cells in the Cdh1 −/− brain, we next looked for Tbr2—an intermediate progenitor cell marker—, Pax6—a neuroepithelial and radial glia cell marker— and active caspase-3 immunostaining in serial sections from the same brain block. As shown in Fig. 6b , active caspase-3 was expressed in both Pax6 + (VZ) and Tbr2 + (basal VZ and SVZ) in the brain cortex. Moreover, neural precursors (Sox2 + /Nestin + cells; Fig. 6c ), but not newly committed neurons (Tuj1 + cells; Supplementary Fig. S2D ), were found to undergo apoptotic cell death. Further, apoptosis was also detected by terminal deoxynucleotidyl transferase dUTP nick end-labelling assay in both Pax6 + and Tbr2 + progenitor cells ( Supplementary Fig. S2E ). Together, these data confirm that Cdh1 is essential for the survival of mouse cortical progenitor cells. 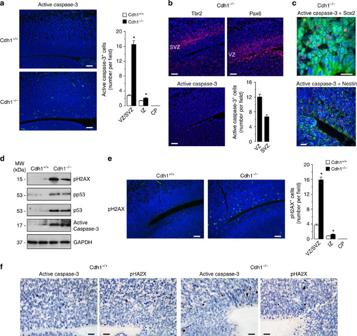Figure 6: Loss of Cdh1 triggers replicative stress and apoptotic cell death in the VZ and SVZ of the cerebral cortex. (a) Fluorescent photomicrographs of both E14.5 Cdh1+/+and Cdh1−/−cerebral cortex immunostained with the apoptotic marker active caspase 3 reveal that Cdh1 deficiency triggers apoptotic cell death in the VZ/SVZ of the brain cortex. Scale bar, 50 μm. (b) Active caspase-3 expression was located in both Pax6+(VZ) and Tbr2+(basal VZ and SVZ) zones. Scale bar, 50 μm. (c) Double labelling revealed that neural precursor cells (Sox2+/Nestin+cells) underwent apoptotic cell death. Scale bar, 20 μm. (d) Western blotting shows that the brain cortex of Cdh1-deficient mice expressed pH2AX and both total (p53) and phosphorylated forms (pp53) of p53, which were absent in Cdh1+/+mice. (e) Immunofluorescent images reveal that replicative stress (pH2AX staining) was found throughout the VZ/SVZ of the Cdh1−/−brain cortex. Scale bar, 50 μm. (f) Replicative stress and activation of capase-3 in the VZ/SVZ of the Cdh1−/−mice were further confirmed by pH2AX and active caspase-3 immunostaining in histological brain sections. Scale bar, 20 μm. Field: 0.25 mm2. *P<0.05 versus Cdh1+/+(Student’st-test;n=4 mice). Data are expressed as mean±s.e.m. Figure 6: Loss of Cdh1 triggers replicative stress and apoptotic cell death in the VZ and SVZ of the cerebral cortex. ( a ) Fluorescent photomicrographs of both E14.5 Cdh1 +/+ and Cdh1 −/− cerebral cortex immunostained with the apoptotic marker active caspase 3 reveal that Cdh1 deficiency triggers apoptotic cell death in the VZ/SVZ of the brain cortex. Scale bar, 50 μm. ( b ) Active caspase-3 expression was located in both Pax6 + (VZ) and Tbr2 + (basal VZ and SVZ) zones. Scale bar, 50 μm. ( c ) Double labelling revealed that neural precursor cells (Sox2 + /Nestin + cells) underwent apoptotic cell death. Scale bar, 20 μm. ( d ) Western blotting shows that the brain cortex of Cdh1-deficient mice expressed pH2AX and both total (p53) and phosphorylated forms (pp53) of p53, which were absent in Cdh1 +/+ mice. ( e ) Immunofluorescent images reveal that replicative stress (pH2AX staining) was found throughout the VZ/SVZ of the Cdh1 −/− brain cortex. Scale bar, 50 μm. ( f ) Replicative stress and activation of capase-3 in the VZ/SVZ of the Cdh1 −/− mice were further confirmed by pH2AX and active caspase-3 immunostaining in histological brain sections. Scale bar, 20 μm. Field: 0.25 mm 2 . * P <0.05 versus Cdh1 +/+ (Student’s t -test; n =4 mice). Data are expressed as mean±s.e.m. Full size image Next, the underlying molecular mechanism involved in Cdh1 loss-induced apoptosis of neural precursor cells was studied. It is known that Cdh1 depletion results in shorter G1 and premature entry into the S phase, that is, when the replicative machinery is not yet ready [25] , [31] , [33] . This triggers a prolonged, unscheduled S-phase progression that results in replicative stress and DNA damage responses [25] , [31] , [33] , leading to activation of the p53 pathway and/or cell death [31] , [33] . The increase in DNA replication ( Figs 2b,c and 5b ) and the induction of apoptosis ( Figs 2g,h and 6a–c ) in Cdh1-null neural precursor cells prompted us to study whether the lack of Cdh1 activated the DNA damage response pathway. As observed in Supplementary Fig. S2F , Cdh1 −/− cortical cells accumulated replicative stress as shown by the high expression of phosphorylated H2AX, a replicative stress marker, after 2 days in culture. Moreover, in good agreement with the fact that replicative stress is coordinated by the ataxia telangiectasia and Rad3-related protein (Atr)-checkpoint kinase1 (Chk1) pathway [34] , loss of Cdh1 increased the phosphorylation of the ATR target Chk1 (pChk1), as well as both total (p53) and phosphorylated forms (pp53) of p53, in cultured cells. Further, pH2AX, pp53, p53 and active caspase-3 were abundantly expressed in the brain cortex of Cdh1 −/− but not in the Cdh1 +/+ mice ( Fig. 6d ). Immunohistochemical images revealed that replicative stress (pH2AX) and activation of caspase-3 (active caspase-3) were found throughout the VZ/SVZ of the Cdh1 −/− brain cortex ( Fig. 6e,f ). Therefore, the lack of Cdh1 induces replicative stress, p53 accumulation and cell death in neural progenitor cells. Given the accumulation of p53 in Cdh1 −/− cerebral cortex, we next tested whether p53 depletion could mitigate cell death in Cdh1 −/− cells. Pharmacological inhibition of p53 in vitro with pifithrin-α prevented the increase in apoptotic death caused by Cdh1 deficiency ( Supplementary Fig. S2F ). Further, knockdown of p53 by RNA interference fully prevented the accumulation of pp53 and p53 in Cdh1 −/− -cultured cells ( Supplementary Fig. S2G ), and abolished the increase in active capase-3 expression ( Supplementary Fig. S2G ) and apoptotic death ( Supplementary Fig. S2H ) caused by Cdh1 deficiency. Strikingly, whereas p53 depletion in Cdh1 +/+ -cultured cells significantly increased cell number, it led to a dramatic loss of viable cells in Cdh1 −/− cultures ( Supplementary Fig. S2I ). Moreover, depletion of p53 did not prevent replicative stress induced by the lack of Cdh1, as shown by the high expression of pH2AX ( Supplementary Fig. S2H ). Thus, the increased growth rates associated with p53 depletion aggravated replicative stress in Cdh1 −/− -cultured cells. To further confirm these in vitro results, we analysed the effect of additionally eliminating p53 in Cdh1-deficient embryos. We found that the cerebral cortex in double-mutant mice (Cdh1 −/− p53 −/− ) was thinner than that in Cdh1 −/− p53 +/+ mice ( Fig. 7a ). BrdU staining revealed pronounced neural progenitor proliferation in cerebral cortex of double-Cdh1, p53-deficient mice ( Fig. 7b ). Lack of p53 totally prevented apoptotic cell death induced by Cdh1 depletion, as shown by the significant decrease in active caspase-3 immunostaining in the VZ/SVZ of Cdh1 −/− p53 −/− mice in comparison with the corresponding areas of Cdh1 −/− p53 +/+ mice ( Fig. 7c ). In contrast, p53 deficiency did not prevent replicative stress induced by Cdh1 loss, as shown by the accumulation of pH2AX-positive cells in the VZ/SVZ of Cdh1 −/− p53 −/− mice ( Fig. 8a ), which was slightly higher to that found in Cdh1 −/− p53 +/+ mice. Moreover, lack of p53 alone (Cdh1 +/+ p53 −/− mice) induced replicative stress in the VZ/SVZ of cerebral cortex ( Fig. 8a ), suggesting a role for p53 in preventing replicative stress in the developing brain. These results corroborate that p53 depletion aggravated replicative stress in Cdh1 −/− cerebral cortex. 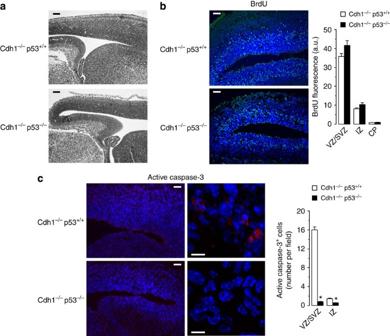Figure 7:Expression of p53 mediates apoptotic cell death of neural progenitor cells in the Cdh1−/−cerebral cortex. (a) Histological staining of brain sections from E14.5 Cdh1−/−p53+/+and Cdh1−/−p53−/−mice. Scale bar, 200 μm. (b) Fluorescent photomicrographs of E14.5 Cdh1−/−p53+/+and Cdh1−/−p53−/−cerebral cortex after immunostaining for a marker of S-phase cells, BrdU. Scale bar, 50 μm. (c) Additional depletion of p53 prevents apoptosis in Cdh1-deficient embryonic brain, as revealed by active caspase 3 immunostaining. Scale bar, 50 μm (left panel), 7 μm (right panel). Field: 0.25 mm2. *P<0.05 versus Cdh1−/−p53+/+(Student’st-test;n=4 mice). Data are expressed as mean±s.e.m. Figure 7: Expression of p53 mediates apoptotic cell death of neural progenitor cells in the Cdh1 −/− cerebral cortex. ( a ) Histological staining of brain sections from E14.5 Cdh1 −/− p53 +/+ and Cdh1 −/− p53 −/− mice. Scale bar, 200 μm. ( b ) Fluorescent photomicrographs of E14.5 Cdh1 −/− p53 +/+ and Cdh1 −/− p53 −/− cerebral cortex after immunostaining for a marker of S-phase cells, BrdU. Scale bar, 50 μm. ( c ) Additional depletion of p53 prevents apoptosis in Cdh1-deficient embryonic brain, as revealed by active caspase 3 immunostaining. Scale bar, 50 μm (left panel), 7 μm (right panel). Field: 0.25 mm 2 . * P <0.05 versus Cdh1 −/− p53 +/+ (Student’s t -test; n =4 mice). Data are expressed as mean±s.e.m. 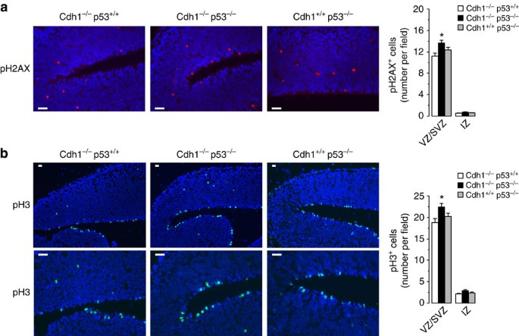Figure 8: Replicative stress induced by Cdh1 loss in the VZ and SVZ of the cerebral cortex is p53 independent. (a) Fluorescent photomicrographs of cerebral cortex from E14.5 Cdh1−/−p53+/+and Cdh1−/−p53−/−mice after immunostaining with pH2AX reveal replicative stress in the VZ/SVZ. Scale bar, 20 μm. (b) Fluorescent photomicrographs of cerebral cortex show that the number of pH3-positive cells in the VZ/SVZ of E14.5 Cdh1−/−p53+/+is further increased by codepletion of p53 (Cdh1−/−p53−/−). Fluorescent photomicrographs reveal (a) replicative stress and (b) increased pH3-positive cells in the VZ/SVZ of Cdh1+/+p53−/−mice. Scale bar, 20 μm. Field: 0.25 mm2. *P<0.05 versus Cdh1−/−p53+/+(analysis of variance;n=4 mice). Data are expressed as mean±s.e.m. Full size image Figure 8: Replicative stress induced by Cdh1 loss in the VZ and SVZ of the cerebral cortex is p53 independent. ( a ) Fluorescent photomicrographs of cerebral cortex from E14.5 Cdh1 −/− p53 +/+ and Cdh1 −/− p53 −/− mice after immunostaining with pH2AX reveal replicative stress in the VZ/SVZ. Scale bar, 20 μm. ( b ) Fluorescent photomicrographs of cerebral cortex show that the number of pH3-positive cells in the VZ/SVZ of E14.5 Cdh1 −/− p53 +/+ is further increased by codepletion of p53 (Cdh1 −/− p53 −/− ). Fluorescent photomicrographs reveal ( a ) replicative stress and ( b ) increased pH3-positive cells in the VZ/SVZ of Cdh1 +/+ p53 −/− mice. Scale bar, 20 μm. Field: 0.25 mm 2 . * P <0.05 versus Cdh1 −/− p53 +/+ (analysis of variance; n =4 mice). Data are expressed as mean±s.e.m. Full size image Finally, we analysed the pattern of phosphorylation of histone H3 (pH3) in brain sections of double-mutant mice to quantify the number of mitotic cells. As shown in Fig. 8b , there was an accumulation of pH3-positive cells in the VS/SVZ of both Cdh1 −/− p53 +/+ and Cdh1 −/− p53 −/− mice, suggesting active M-phase cells. The number of pH3-positive cells was higher in cerebral cortex of Cdh1 −/− p53 −/− mice when compared with the corresponding area in the Cdh1 −/− p53 +/+ mice. Further the accumulation of pH3-positive cells was also observed in the VZ/SVZ of the p53-knockout mice ( Fig. 8b ). Thus, depletion of p53 increases the number of mitotic cells in the VZ/SVZ of Cdh1 −/− mice, as described for replicative stress. In summary, loss of Cdh1 causes aberrant cell cycle progression in neural progenitor cells and delays their exit from the cell cycle to generate post-mitotic neurons. In turn, this causes replicative stress triggering p53-dependent apoptotic death in neural progenitors of the VZ and SVZ of the cerebral cortex. Further, p53 depletion enhances replicative stress in neural precursor cells from Cdh1 −/− brain, which results in the aggravation of the cortical size reduction. Here we show that the E3 ubiquitin ligase APC/C-Cdh1 coordinates the cell cycle exit with the initiation of the differentiation process of neural progenitor cells. Genetic elimination of the APC/C activator Cdh1 dramatically delays neural progenitor cells exit from the cell cycle, leading to replicative stress, p53-mediated apoptotic death and significant reduction of the cortical size. We describe that neuronal differentiation in vitro implied the rapid degradation of the APC/C-Cdh1 substrate F-box protein Skp2, leading to the stabilization of the Cdk inhibitor p27, ultimately resulting in cell cycle exit. Accordingly, differentiation of rat pheochromocytoma cell line PC12 (ref. 35 ) and human neuroblastoma cell line SH-SY5Y (ref. 30 ) to a neuronal phenotype requires Skp2 elimination and p27 stabilization. Further, APC/C-Cdh1-mediated Skp2 degradation is required during myogenesis [36] and lens epithelial differentiation [37] . All these data pose the APC/C-Cdh1-Skp2-p27 axis as a well-conserved signalling pathway in cell differentiation in vitro . We also reveal the critical importance of the phosphorylation status of Cdh1 on neuronal differentiation and survival in vitro . We found that the progressive increase in APC/C-Cdh1 activity correlated with the decrease in Cdk1 activity along the differentiation process of neurons. This is consistent with the notion that APC/C-Cdh1, by promoting cyclin B1 degradation [15] , [38] , inhibits Cdk1 activity to support the neuronal phenotype. We also found that non-phosphorylated Cdh1 was required for the functional activity of APC/C-Cdh1 in promoting neuronal differentiation. This was further confirmed by ectopically expressing a phospho-mimetic and a non-phosphorylatable form of Cdh1, which, respectively, either delayed or accelerated cell cycle exit and neurite extension of cultured progenitor cells. Besides the negative effect on neuronal differentiation progress, failure to dephosphorylate Cdh1 also resulted in the apoptotic death of progenitor cells. Together, these results indicate that dephosphorylated Cdh1 keeps APC/C-Cdh1 functionally active to support both the differentiation and the survival of neural progenitor cells in vitro . Further, the effects caused by the inhibitory phosphorylation of Cdh1 are fully replicated by the PP2A blocker okadaic acid. Recent data indicating that PR61/B'δ (a PP2A subunit highly expressed in neural tissues)-null mice show neurological problems [39] highlight the importance of protein phosphatases in neural diseases. In view of the fact that phosphorylated Cdh1 is a PP2A substrate [40] , it would be very interesting to decipher whether the dysfunctional PP2A mice [39] , by impeding Cdh1 dephosphorylation during neuronal differentiation in the early embryonic period, mimic the neurodevelopmental problems observed in the Cdh1 −/− mice. The implication of Cdh1 in the in vitro neuronal differentiation process of progenitor cells was further validated using an embryo-restricted Cdh1-knockout mouse model [25] . Cortical cells of the Cdh1 −/− embryos lack the ability to acquire a typical neuronal phenotype in culture, as assessed by Map2 protein abundance, BrdU incorporation, cell cycle protein expression and neurite extension. In accordance with previous results [25] , [30] , [31] , we also found that Cdh1 loss delays cell cycle exit, shortens G1 phase and prolongs S and G2/M phases. Moreover, we show that cerebral cortex of E14.5 Cdh1 −/− mice showed a reduction of newly differentiated neurons at the expense of increased DNA replication of progenitor cells. This is in good agreement with previous results showing fewer cortical neurons and reduced cortical size as a consequence of experimental prolongation of cell cycle of neural precursors [10] , [41] . In our Cdh1 −/− mice, the lengths of the VZ/SVZ are increased, whereas those of the IZ and CP layers of the cortex are reduced, leading to reduced cerebral cortical size, which is a phenotype compatible with MCPH [42] . It is interesting to note that genetic defects in DNA damage response lead to human MCPH syndromes, such as ATR Seckel syndrome, caused by mutations in the gene encoding the ATR protein [43] , and primary MCPH caused by mutations in MCPH1 (ref. 44 ), indicating that MCPH may be caused by alterations of neuronal progenitors in response to DNA damage [45] , [46] . We previously reported [25] that Cdh1 −/− cells show premature entry into S phase and replicative defects. Conversely, results from other laboratories showed that Cdh1 depletion initiates aberrant DNA replication, triggering a p53-mediated response to DNA damage in cultured human cells [33] , [31] . Here we further demonstrate that loss of Cdh1 in vivo triggers cyclin B1 accumulation and replicative stress in the cerebral cortex. In this sense, high levels of cyclin B1-CDK1 activity prevent the assembly of origins of replication and the efficient timing of S phase [15] , which could lead to DNA replicative stress. In turn, this would activate a p53-mediated apoptotic death-signalling pathway in neural progenitor cells in the VZ/SVZ resulting in reduced neurogenesis and MCPH in Cdh1-deficient mice. Interestingly, knockdown of p53 in vitro , and genetic deletion of p53 in vivo , abolished apoptotic cell death. On the contrary, p53 loss increases neural progenitors loss in vitro and aggravates MCPH caused by Cdh1 deficiency in vivo . Further, depletion of p53 enhances Cdh1 −/− -mediated neural progenitor proliferation, as revealed by BrdU and pH3 staining, which triggers the increase in the amount of replicative stress in the cerebral cortex. Taken together, these findings indicate that p53 mediates the apoptotic death in the brain but aggravates replication stress and MCPH phenotypes of the Cdh1 −/− mice. In this context, mutations that promote cell proliferation further potentiate replicative stress that, if sufficiently high, compromises cell viability [47] , [48] , as we observed in the Cdh1 −/− mice. Recently, Murga et al. [47] described that p53 loss increases replicative stress leading to aggravation of neurodevelopmental damage and MCPH phenotypes in a murine model of the human ATR Seckel syndrome characterized by a severe deficiency in ATR. In this context, the increased amount of replicative stress generated by p53 loss in the ATR-deficient mice also increases the amount of cell eliminated by apoptosis during embryogenesis [47] . Similarly, loss of Chk1 leads to p53-independent cell death in zebrafish [49] . We thus speculate that a similar pathway might be occurring in the Cdh1 −/− p53 −/− -mutant mice. Alternatively, the accumulated pool of neural precursor cells in the VZ/SVZ of Cdh1 −/− cerebral cortex could be suggestive of a migration defect. Recently, Qin and Zhang [50] have described that downregulation of the APC/C-Cdh1 target KLF4 (ref. 51 ) is essential for normal neurogenesis. Similarly, neural progenitor cells with high expression of KLF4 fail to migrate and develop into neurons [50] . Future studies would be needed to fully understand the role of Cdh1 on neuronal migration during brain development. In conclusion, here we describe that loss of Cdh1 reduces the length of the G1 phase and increases S-phase duration in neural precursor cells, which generates replicative stress, triggering apoptotic death of neural precursor cells. Consequently, neurogenesis is severely affected leading to the shortening of the cerebral cortex and relative brain size, compatible with microencephaly ( Supplementary Fig. S3 ). In addition, we reveal that p53 wholly account for the apoptotic cell death of neural progenitors. These results demonstrate that APC/C-Cdh1 coordinates cortical neurogenesis and size, thus posing Cdh1 in the molecular pathogenesis of congenital neurodevelopmental disorders, such as MCPH. Sox2-Cre-mediated Cdh1 conditional knockout mice The Cdh1 lox/lox -targeted mouse model was generated by flanking exons 2 and 3 of the murine Fzr1 locus with loxP sequences [25] . To obtain Cdh1-deficient mice ( Cdh1 − / Δ ; Sox2-Cre +/T , referred as Cdh1 −/− ), a transgenic strain expressing Cre in embryonic but not in extra-embryonic tissues (Sox2-Cre) was used [29] . We also utilized Cdh1 +/ Δ ; Sox2-Cre +/T (referred as Cdh1 −/+ ) and Cdh1 +/ lox ; Sox2-Cre +/+ (referred as Cdh1 +/+ ) mouse embryos. To generate embryos deficient for p53 and Cdh1, we set up crosses between 2–3-month-old Cdh1 lox/lox ; Sox2-Cre +/+ ; p53 +/− female mice and 2–5 month Cdh1 +/− ; Sox2-Cre +/T ; p53 −/− male mice. For BrdU incorporation in 14.5-day-old embryos, timed pregnant females were administered BrdU at 50 mg kg −1 of body weight by intraperitoneal injection. All animals were maintained in a mixed 129/Sv (25%) × CD1 (25%) × C57BL/6J (50%) background. All animals used in this work were obtained from the Animal Experimentation Unit of the University of Salamanca, in accordance with Spanish legislation (RD 1201/2005) under licence from the Spanish Ministry of Science and Innovation. Mice were housed under standard conditions in the pathogen-free animal facility of the University of Salamanca (Salamanca, Spain) following the animal care standards of the institution. Animal experiments were approved by the Bioethics Committee of the University of Salamanca. Cell culture treatments and transfections Primary cultures of cortical neurons were prepared from E14.5 mouse embryo cortices. Cells were seeded at 2.0 × 10 5 cells cm −2 in DMEM (Sigma, Madrid, Spain) supplemented with 10% (v/v) FCS (Roche Diagnostics, Heidelberg, Germany) and incubated at 37 °C in a humidified 5% CO 2 -containing atmosphere. At 4 h after plating, the medium was replaced with Neurobasal medium (Invitrogen, Madrid, Spain) supplemented with 2% B27 (Invitrogen) and glutamine 4 mM (Invitrogen). When indicated, medium contained the phosphatase inhibitor okadaic acid (10 nM) [52] or exposed to the specific inhibitor of p53-mediated transcriptional activation, pifithrin-α (10 nM) [53] . Cells were transfected 4 h after plating with plasmid DNA or short interfering RNA (siRNA) using Lipofectamine2000 (Invitrogen). hEmi1 was used to inhibit the APC/C complex by co-transfecting cells with pCS2-hEmi1 (generously donated by Dr Peter Jackson, Stanford University School of Medicine, Stanford, CA) plus pGFP (Clontech Laboratories Inc., Palo Alto, CA) to identify transfected (green fluorescent protein; GFP + cells) cells, and control transfections were carried out with a truncated form of hEmi1 carrying a deletion of the zinc-binding region that causes loss of function (pCS2-Myc5-hEmi1DZBR, generously donated by Dr Peter Jackson). Human full-length Cdh1 complementary DNA was a generous gift of Dr J Pines (Gurdon Institute, University of Cambridge, UK) and was used to obtain the Ser-40, Thr-121 and Ser-163 triple alanine (Cdh1-A) or aspartate (Cdh1-P) Cdh1 mutants using the QuikChange XL site directed mutagenesis kit (Stratagene, La Jolla, CA, USA). Residues were mutated either to Ala (Cdh1-A; to block phosphorylation) or to Asp (Cdh1-D; to mimic a phosphorylated status) [54] . Cells were transfected with the pIRES2-EGFP mammalian expression vector (Invitrogen) co-expressing the enhanced GFP and either the full-length wild type or mutant forms of Cdh1 (ref. 54 ). Depletion of p53 was performed by siRNA (5′-CCACUUGAUGGAGAGUAUUUU-3′) [55] ; siRNA against luciferase was used for control transfections [38] . For plasmids, the transfection efficiencies in neurons were, approximately, 7%, as judged by the proportion of GFP + neurons versus total number of neurons (as evidenced by flow cytometry analysis); for siRNA, the transfection efficiencies were >90%, as judged by the level of protein knockdown shown in the Supplementary Fig. S2F . BrdU incorporation into DNA and cell cycle phase percentage were determined by flow cytometry. This was achieved after 3 h of incubation with 10 mg ml −1 BrdU using the APC BrdU Flow Kit (BD Biosciences), following the manufacturer’s instructions [30] . When cell phenotype was studied, cells were fixed and permeabilized using the Fix&Perm kit from Caltag (Invitrogen) and were stained with Nestin-APC and Tuj1-PE (BD Biosciences), according to the protocol included in the technical data sheet. The percentage of cells expressing Nestin and Tuj1 were quantified by flow cytometry. Western blotting Cells were lysed in buffer containing 1% SDS, 2 mM EDTA, 150 mM NaCl, 12,5 mM Na 2 HPO 4 and 1% Triton X-100, supplemented with phosphatase inhibitors (1 mM Na 3 VO 4 and 50 mM NaF) and protease inhibitors (100 μM phenylmethylsulfonyl fluoride, 50 μg ml −1 anti-papain, 50 μg ml −1 pepstatin, 50 μg ml −1 amastatin, 50 μg ml −1 leupeptin, 50 μg ml −1 bestatin and 50 μg ml −1 soybean trypsin inhibitor) and boiled for 5 min. Protein concentrations were determined with the BCA Protein Assay kit (Thermo Fisher Scientific). Extracts were centrifuged at 13,000 g for 5 min at 4 °C. Aliquots of lysates (20–50 μg protein) were subjected to SDS–polyacrylamide gel electrophoresis and blotted with anti-Map2 (1:200)(ab32454, Abcam), anti-phosphoserine (1:1,000) (ab9332, Abcam), anti-Cdh1 (1/20) (AR38, a generous gift from Dr J Gannon, Clare Hall Laboratories, Cancer Research UK), anti-Skp2 (1:200) (32-3,400, Zymed), anti-p27 (1:1,000) (554069, BD Biosciences), anti-Cdk1 (1:250) (610037, BD Biosciences), anti-cyclin B1 (1:100) (554176, BD Biosciences), anti-p53 (1:100) (554157, BD Biosciences), anti-pp53 (1:500) (Ser15; 9286, Cell Signaling), anti-pH2AX (1:250) (Ser139, 05-6360, Upstate), anti-active caspase 3 (1:500) (Asp175, 9661 Cell Signaling), anti-pChk1 (1:500) (Ser317, 2344 Cell Signaling) or anti-GAPDH (1:40,000) (glyceraldehyde-3-phosphate dehydrogenase; Sigma) overnight at 4 °C. Signal detection was performed with an enhanced chemiluminescence detection kit (Thermo Fisher Scientific). Full blots and gel scans are included in Supplementary Fig. S4 . Cdk1 kinase assay Cells were lysed in ice-cold buffer containing 50 mM Tris (pH 7.5), 150 mM NaCl, 10 mM EDTA, 2 mM EGTA, 1% NP-40, supplemented with the phosphatase and protease inhibitors cited above. After clearing debris by centrifugation, extracts (200 mg protein) were incubated with anti-Cdk1 (2 mg) for 4 h at 4 °C, followed by the addition of 30 ml of protein A-agarose (GE Healthcare Life Sciences) for 2 h at 4 °C. Immunoprecipitates were washed four times in lysis buffer and resuspended in kinase buffer (20 mM Tris pH 7.6, 20 mM MgCl 2 , 2mM MnCl 2 , 1 mM EDTA, 1 mM EGTA and 0.1 mM dithiothreitol) containing 20 mM ATP, 10 mCi of [γ- 32 P]ATP and histone H1 (50 mg ml −1 ; Sigma). Samples were subjected to SDS–polyacrylamide gel (12%) electrophoresis and transferred proteins were visualized by autoradiography or blotted with anti-Cdk1 (1:250) (610037, BD Biosciences). APC/C ubiquitin ligase activity Active APC/C was immunoprecipitated from cell nuclear extracts using monoclonal anti-APC3 antibody (10 μg) (610455, BD Biosciences) and immobilized on Dynabeads Protein A (Invitrogen). For ubiquitination assays, immunoprecipitates were incubated at 37 °C in 10 μl of buffer (0.1 M KCl, 2.5 mM MgCl 2 , 2 mM ATP, 7.5 μg ubiquitin, 0.3 mM dithiothreitol, 135 mM MG132, 1 mM ubiquitin aldehyde, 2.5 mM His-UbcH10 and 2.5 μM UbcH5a in 20 mM Tris–HCl, pH 7.5) containing 2.5 μl of APC/C beads and 1 μl of [ 35 S]cyclin B1. Reactions were stopped at the indicated time points with SDS sample buffer, mixtures resolved by SDS–polyacrylamide gel electrophoresis and visualized by phosphorimaging [54] . Flow cytometric detection of apoptotic cell death Neurons were carefully detached from the plates using 1 mM EDTA (tetrasodium salt) in PBS (pH 7.4) and were stained with annexin V-APC and 7-AAD in binding buffer (100 mM HEPES, 140 mM NaCl, 2.5 mM CaCl 2 ) to determine quantitatively the percentage of apoptotic neurons by flow cytometry. Cells were stained with annexin V-APC and 7-AAD in binding buffer (100 mM HEPES, 140 mM NaCl, 2.5 mM CaCl2), according to the manufacturer’s instructions, and 3 × 10 5 cells were analysed, in four replicates per condition, on a FACScalibur flow cytometer (15 mW argon ion laser tuned at 488 nm; CellQuest software, BD Biosciences). Transfected (identified by GFP+ fluorescence) cell population were analysed, and the annexin V-APC-stained cells that were 7AAD negative were considered to be apoptotic. Flow cytometric detection of active caspase-3 Active caspase-3 was detected using the ApoActive3 Kit (Bachem, San Carlos, CA, USA), following the manufacturer’s instructions. After detaching cells with 1 mM EDTA (tetrasodium salt) and centrifugation, cell pellets were fixed during 20 min, resuspended in PBS+2% BSA and incubated for 1 h with 1 × rabbit anti-caspase 3. Cells were then incubated with 1:500 anti-rabbit Cy3 (Jackson ImmunoResearch) for 1 h. Between each step, cells were washed with either PBS (until labelling of samples) or PBS+1% BSA and resuspended in PBS+1% BSA before analysis by flow cytometry (tuned at 488 nm; CellQuest software, BD Biosciences) [53] . When cell phenotype was studied, cells were fixed and permeabilized using the Fix&Perm kit from Caltag (Invitrogen) and were stained with active caspase-3-fluorescein isothiocyanate (1:10) (560901), Nestin-APC (1:10) (560393) and Tuj1-PE (1:10) (560381) (BD Biosciences), according to the protocol included in the technical data sheet. The percentage of active caspase-3 + cells expressing Nestin and Tuj1 were quantified by flow cytometry. Immunohistochemistry Timed murine embryos were harvested from pregnant dams according to animal care standards of the University of Salamanca. The embryo heads were fixed with 4% (w/v) paraformaldehyde, 0.2% (w/v) picric acid in 0.1 M phosphate buffer pH 7.4 (ref. 56 ) for 10 days at 4 °C. Brains were removed from the skull, post-fixed for an additional day and sagittally dissected out in two parts. Brain blocks were rinsed successively for 10 min, 30 min and 2 h with 0.1 M PBS (pH 7.4), and immersed in sucrose/PBS with concentrations of 20 and 30% sequentially until they sank. After cryoprotection, tissues were embedded in Optimal cutting temperature compound (OCT) (catalogue #4583; Thermo Fisher Scientific) and frozen with liquid nitrogen. Finally, brains were sectioned in the sagittal plane on a cryostat at 20 μm and mounted onto Superfrost Plus slides (Thermo Fisher Scientific). Sagittal sections containing the entire cortex were selected, rinsed twice in 0.1 M PBS and single- or double-labelled with the corresponding antibodies diluted in blocking solution (0.2% Triton X-100 and 5% normal goat serum in 0.1 M PBS) for 72 h at 4 °C, followed by secondary antibody labelling for 2 h at room temperature and 4',6-diamidino-2-phenylindole staining (0.5 μg ml −1 4',6-diamidino-2-phenylindole in PBS) for 10 min. After each step, sections were carefully rinsed three times for 10 min each in PBS. Sections were mounted with Fluoromount (Sigma) aqueous mounting medium and examined on a microscope (Nikon Inverted 13 microscope Eclipse Ti-E) equipped with a pre-centred fibre illuminator (Nikon Intensilight C-HGFI) and Black and White charge-coupled device digital camera (Hamamatsu ORCAER), or on a confocal microscope (TCS SP2; Leica, Mannheim, Germany). For Nestin, Ki67 and active caspase-3 staining, an antigen retrieval procedure was required [57] . For BrdU staining, sections were pre-treated with DNAse (10 μg per slide) at 37 °C for 1 h and washed three times in 0.1 M phosphate buffer for 5 min. The primary antibodies used were the following: rabbit monoclonal anti-Ki67(1/200) (RM-9106, NeoMarkers), mouse monoclonal anti-BrdU (1:500) (RPN2012, Amersham), rabbit polyclonal anti-neuron-specific beta III Tubulin-neuronal marker (1:500) (Tuj 1, ab18207, Abcam), rabbit polyclonal anti-Map2-neuronal marker (1:500) (Map2, ab11267 Abcam), mouse monoclonal anti-nestin (1:500) (556309, BD Pharmingen), rabbit polyclonal anti-Pax6 (1:250) (PRB-278P, Covance Research Products Inc), rabbit polyclonal anti-Tbr2 (1:250) (ab23345, Abcam), mouse monoclonal anti-Sox2 (1:50) (97959, Abcam) and rabbit polyclonal anti-active caspase-3 (1:50) (9661S, Asp175, Cell Signaling). Secondary antibodies were Alexa 568-conjugated goat anti-rabbit (1:500), Alexa 488-conjugated goat anti-rabbit (1:500) and Alexa 594-conjugated goat anti-mouse (1:500) (Molecular Probes, Invitrogen), Cy2-conjugated affiniPure goat anti-mouse (1:500) and Cy3-conjugated affiniPure goat anti-rabbit (1:500) (Jackson ImmunoResearch). Occasionally, embryos were fixed in 10%-buffered formalin (Sigma) and embedded in paraffin wax. Sections of 3 or 5 μm thickness were stained with haematoxylin and eosin for histological examination or processed for immunohistochemical analysis using specific antibodies against active caspase-3 (1:50) (9661S, Asp175, Cell Signaling), pH2AX (1:250) (clonJBW301, Ser139, 16-193, Millipore) and pH3 (1:100) (06-570, Cell Signalling). Terminal deoxynucleotidyl transferase dUTP nick end-labelling assay was performed following the manufacturer’s protocol (3333566, Roche Diagnostics). Immunohistochemistry digital images (RGB images) were used for fluorescence quantification, using the NIH image-processing package ImageJ (ImageJ 1.43n; Java 1.6.0_26[64-bit]). Mean fluorescence values were measured in the whole-image area or in the VZ/SVZ, IZ or CP area defined in Fig. 4 . The pixel intensities ranged from 0 (black) to 255 (white). Fluorescence background was measured and subtracted. Values are mean±s.e.m. from 20 measurements from 4 different brain sections and are expressed as arbitrary units (a.u.) of fluorescence. Statistical analysis Measurements from individual cultures were always performed in quadruplicate. The results are expressed as mean±s.e.m. values for four different culture preparations. For the in vivo experiments, we used four to six animals per condition. Statistical analysis of the results was performed by one-way analysis of variance, followed by the least significant difference multiple range test or by the Student’s t -test for comparisons between two groups of values. In all cases, P <0.05 was considered significant. How to cite this article: Delgado-Esteban, M. et al. APC/C-Cdh1 coordinates neurogenesis and cortical size during development. Nat. Commun. 4:2879 doi: 10.1038/ncomms3879 (2013).